Exploring the MHC-peptide matrix of central tolerance in the human thymus Ever since it was discovered that central tolerance to self is imposed on developing T cells in the thymus through their interaction with self-peptide major histocompatibility complexes on thymic antigen-presenting cells, immunologists have speculated about the nature of these peptides, particularly in humans. Here, to shed light on the so-far unknown human thymic peptide repertoire, we analyse peptides eluted from isolated thymic dendritic cells, dendritic cell-depleted antigen-presenting cells and whole thymus. Bioinformatic analysis of the 842 identified natural major histocompatibility complex I and II ligands reveals significant cross-talk between major histocompatibility complex-class I and II pathways and differences in source protein representation between individuals as well as different antigen-presenting cells. Furthermore, several autoimmune- and tumour-related peptides, from enolase and vimentin for example, are presented in the healthy thymus. 302 peptides are directly derived from negatively selecting dendritic cells, thus providing the first global view of the peptide matrix in the human thymus that imposes self-tolerance in vivo . A functional immune system must be able to effectively recognize and fight pathogens while staying tolerant to the body’s own components. This is achieved by central and peripheral tolerance mechanisms. Central tolerance to self is imposed on T cells during their development in the thymus, where they are educated to be self-referential, recognizing peptides bound to self-major histocompatibility complex (MHC) molecules, as well as self-tolerant, meaning that they remain unresponsive to self-peptides displayed on the very same MHC molecules [1] , [2] . In order to fulfil both criteria, the αβ T cells must pass through two major checkpoints in their development, which are controlled by antigen-presenting cells (APCs) in distinct thymic microenvironments. These APC comprise cortical (cTECs) and medullary thymic epithelial cells (mTECs), as well as both resident and immigrant dendritic cells (DCs). During development, thymocytes must rearrange their genes in order to express a functional T-cell receptor (TCR) that can successfully interact with self-peptide-MHC ligands on cTEC, from which they will then receive a survival signal (positive selection). Positively selected thymocytes migrate into the thymic medulla, where they interact with self-peptide–MHC complexes displayed by mTECs and DCs. T cells expressing a high affinity TCR for these complexes will be negatively selected and undergo apoptosis. Only T cells with a low/intermediate affinity TCR for self-peptides will be allowed to leave the thymus as naive or regulatory T cells [1] , [2] . If a T cell that strongly recognizes self-peptides fails to be deleted, for example, because the corresponding self-protein is not expressed in the thymus or the epitope is destroyed during antigen processing, autoreactive T cells can escape into the periphery, where they can be activated and cause autoimmune disease [3] . Therefore, the interaction between the TCR of developing thymocytes and the MHC peptide ligandome of distinct thymic APCs is crucial for shaping the T-cell repertoire and central tolerance. Myeloid DCs (mDCs) in the thymus were the first cells discovered to be responsible for deletion of autoreactive T cells in the thymus and are crucial for maintaining tolerance to self [4] , [5] . Although, in contrast to mTECs, they are not specialized in expressing tissue-specific antigens such as proinsulin, they can efficiently capture these from mTECs and present them to developing T cells, inducing their deletion, a process that involves autoimmune regulator expression (AIRE) in mTECs [6] , [7] . A role of plasmacytoid DCs (pDCs) in negative selection has only been described very recently [8] and thymic B cells might also be able to contribute to negative selection [9] . Although so far there is no direct proof that the different subsets of thymic APCs present different sets of peptides, there are two strong lines of indirect evidence supporting this notion. First, the different APCs express different sets of self-proteins. In addition to constitutively expressed house-keeping proteins and cell-type-specific proteins, mTECs express tissue-restricted antigens such as insulin under the control of the AIRE transcription factor [10] , [11] . Also, blood-born mDCs and pDCs can import peripheral antigens into the thymus where they delete self-reactive thymocytes [8] , [12] . Second, both the MHC I and II antigen-processing machinery differs between different thymic APCs, which should influence the epitopes that are generated [13] , [14] , [15] , [16] . The different APCs thus contribute to the diversity of the ‘immunological self’ displayed in the thymus shaping the characteristics of the mature T-cell repertoire of each individual. Our current knowledge regarding the self-peptide repertoire in the thymus derives mostly from studies in TCR transgenic mouse models, where expression of a particular antigen is a prerequisite for positive/negative selection. However, none of these studies provides evidence that the respective peptides actually contribute to negative selection under physiological conditions. In the early nineties, Marrack et al. [17] successfully identified ~20 MHC II-bound peptides in pooled thymi of several hundred mice and a few natural ligands for positive selection of mouse OT-I cells are known [18] , [19] . More recently, another group has eluted peptides from whole-mouse thymus, using bioinformatics to narrow down on likely MHC I ligands [20] . In humans, presentation of an epitope from proinsulin on thymic DCs has been reported using monoclonal antibodies [21] , but beyond this, the human thymic peptide repertoire is unknown. In this work we set out to explore the human thymus MHC ligandome. We describe an in depth analysis of the peptide repertoire presented by both MHC class I and class II molecules in the healthy human thymus, both for whole thymus as well as isolated thymic mDCs. In summary, we here present the first data on naturally occurring peptides on which human T cells are selected under physiological conditions, including peptides from DCs which are responsible for deletion of autoreactive T cells. Identification of peptides presented by thymic APCs To address the question which peptides are naturally presented to developing thymocytes to induce negative selection under physiological conditions in humans, we analysed peptides eluted from both MHC I (pan-class I human leucocyte antigen; HLA) and II (HLA–DR) complexes from isolated thymic mDCs by mass spectrometry and compared them with the repertoire of the MHC-bound peptides eluted from cells of the APC-enriched, mDC-depleted (containing pDCs, TECs and other thymic APCs, that is, ligands for both positive and negative selection) as well as whole-thymus fractions ( Fig. 1 ). 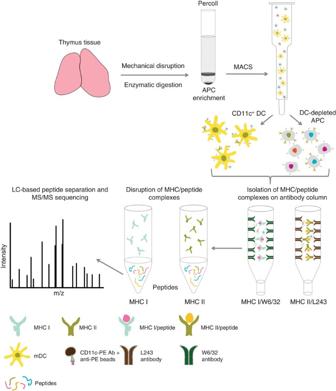Figure 1: Workflow diagram for the isolation of MHC I and MHC II ligands from CD11c+mDC and the DC depleted, APC-enriched fractions.  Figure 1: Workflow diagram for the isolation of MHC I and MHC II ligands from CD11c + mDC and the DC depleted, APC-enriched fractions. Full size image One major challenge for MS-based analysis of peptides presented by thymic APCs is their low frequency and their purification in sufficient numbers to allow ligandome analysis. Typically, the number of cells needed for such experiments is in the order of 10 8 , limiting the possibilities for analysis of primary purified cell types. In our experiments, we identified a total of 842 peptides from the different cell preparations of the eight individual thymi investigated, of which 621 were eluted from MHC I and 221 from MHC II molecules. In the individual mDC preparations, we successfully identified up to 90 peptide sequences eluted from MHC I molecules and up to 48 from MHC II from as little as 30 × 10 6 cells from four different donors ( Table 1 ). Complete lists of the peptide sequences obtained from the different samples and their source proteins are given in Supplementary Data 1 . Table 1 MHC I and MHC II ligands identified on thymic CD11c + dendritic cells of individual donors. Full size table Cross-talk between MHC I and MHC II pathways Peptides presented by MHC I and II derive from different cellular compartments. Typically, nuclear and cytosolic proteins are presented by MHC I, while proteins that are present in the vesicular compartments or the cell membrane or are taken up from the extracellular environment are presented by MHC II molecules. However, especially in professional APCs, there is considerable cross-talk between those two pathways [22] . Mechanisms by which cytosolic/nuclear proteins gain access to the MHC II pathway include autophagy and uptake of apoptotic cells [23] , [24] . Vice versa , proteins or peptides can shuttle out of the lysosome into the cytosol and thus gain access to the MHC I pathway [22] . In addition to this intracellular cross-talk, DCs may take up antigens from other cells such as mTECs, further broadening their peptide repertoire [25] , [26] . To gain insight into the origin of the presented peptides as well as the dynamics of antigenic cross-talk between MHC presentation pathways in thymic mDCs and non-mDC APCs, we performed automated database analysis supplemented by manual annotation of the source proteins and their subcellular localization. Depending on their topological origin, proteins were assigned either to the classical MHC class I (cytosolic, nuclear) or the MHC class II (extracellular, secretory, endocytic, and cell membrane) pathway, the mitochondrial and the ER compartment ( Fig. 2a ). As expected, the majority of MHC I ligands presented by both DCs and non-DC APCs derived from cytosolic/nuclear proteins, that normally do not intersect the endocytic compartment, such as histones, cytoskeletal proteins (actin, tubulin and fascin), metabolic enzymes (protein phosphatase 1, hydroxypyruvate reductase), and cytosolic chaperones (heat shock proteins). MHC class II-bound peptides originated from proteins present in different cellular compartments, including the extracellular milieu, the plasma membrane and the vesicular compartment with membrane proteins being the most abundant peptide generators (mostly from MHC class II proteins) in agreement with previous studies with other cell types [24] . A substantial number of MHC II presented peptides originated from blood or serum proteins, such as serum albumin, haemoglobin and apolipoprotein A2, providing direct evidence that thymic DCs sample the blood stream. 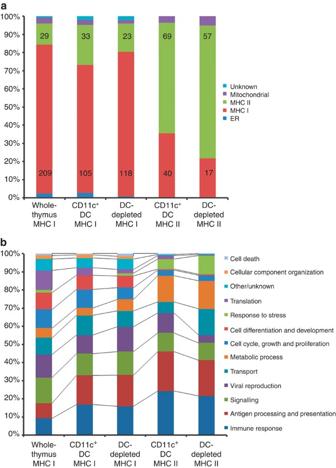Figure 2: MHC pathway assignment and functional categorization of the identified source proteins isolated from the different thymic sample preparations. The cellular localization (a) and biological processes (b) of the protein categories represented graphically as percentages are based onn=the number of the individual proteins identified in each thymic APC preparation. Figure 2: MHC pathway assignment and functional categorization of the identified source proteins isolated from the different thymic sample preparations. The cellular localization ( a ) and biological processes ( b ) of the protein categories represented graphically as percentages are based on n =the number of the individual proteins identified in each thymic APC preparation. Full size image Interestingly, a considerable fraction of the MHC II ligands derived from source proteins localized to the cytosol or nucleus (35.4% in DCs and 21.8% in non-DCs), which are topologically separated from the MHC class II pathway. Similarly, 22.4% of MHC I ligands on DCs derived from the vesicular/extracellular compartment (compared with 15.5% in the DC-depleted fraction and 11.4% in the complete thymus samples). Peripheral DCs are highly efficient at cross-presenting endocytosed antigens on MHC I and cytosolic/nuclear antigens on MHC II. It is therefore crucial to induce central tolerance also to cross-presented self-proteins. The high degree of cross-talk between the two pathways that we observe in thymic DCs, as well as to a lesser extent in the DC-depleted fraction, reflects this need to avoid peripheral autoimmune responses by deleting T cells that recognize cross-presented self-proteins. A recent study has underscored the importance of autophagy for MHC II presentation during central tolerance induction. In mice, genetic interference with autophagy leads to an altered selection of certain CD4 + T-cell specificities that give rise to an autoreactive T-cell repertoire [27] . Most of the studies so far have addressed the in vivo relevance of autophagy mainly in TECs, and not thymic DCs, but in peripheral DCs autophagosomes have been shown to fuse with the MHC II loading compartment [23] . Our peptide data show considerable presentation of peptides derived from nuclear/cytosolic as well as some mitochondrial proteins on MHC class II by thymic mDCs, suggesting a role for autophagy in MHC II ligands sampling in these cells. Alternatively, these proteins could enter the MHC II pathway by uptake from other cells such as apoptotic thymocytes or live/dying mTECs [7] , [28] , [29] or transfer of peptide–MHC complexes from mTECs [30] . Nature of DC-presented peptides Analysis of the biological processes associated with the peptides’ source proteins revealed a prominent fraction of proteins participating in ‘immune response’ and ‘antigen processing/presentation’, biological functions reflecting the nature of the thymus as an immune organ ( Fig. 2b ). The most highly represented class of proteins in these groups were HLA molecules and, not surprisingly, their presence was more pronounced in the DC and DC-depleted samples (enriched for other thymic APCs), compared with whole-thymus samples. Most of the remaining class I and II natural ligands derive from house-keeping proteins (signalling, translation, metabolism, cell cycle and proliferation). Interestingly, peptides derived from proteins associated with metabolic processes are preferentially presented on MHC class II molecules, and peptides derived from proteins involved in cell cycle, growth, proliferation and differentiation are more abundantly presented on MHC class I molecules. The explanation for the preferential presentation of peptides derived from proteins involved in these processes by MHC I is that in these groups the majority of peptides derive from nuclear and cytosolic proteins involved in maintaining cellular structure (for example, the cytoskeleton) and transcription. These are typically degraded by the proteasome and presented via the classical MHC I pathway [22] . A closer look at the metabolic processes-associated proteins revealed that many of the MHC II-bound identified peptides in this group derived from cytosolic proteins. The sources of these peptides included a considerable number of long-lived constitutive metabolic enzymes like glyceraldehyde 3-phosphate dehydrogenase and phosphoglycerate kinase 1. Interestingly, long-lived proteins have been suggested to be disposed by autophagic rather than proteasomal protein degradation [31] . Autophagic degradation of cellular material has been shown to significantly contribute to the peptide pool presented by MHC II (refs 23 , 24 ). In agreement with our results and in support of this idea, glyceraldehyde 3-phosphate dehydrogenase was previously identified as a source of natural MHC class II, but not class I ligands [24] , [32] . Hence, autophagic degradation of long-lived metabolic proteins might explain why these cytosolic proteins are presented by MHC class II rather than class I. The observed wide cellular functional distribution of proteins reflects the wide range of proteins that serve as a matrix for self-protein presentation in the thymus. Peptides differ between individuals and APC It has been suggested that different types of thymic APC present different non-overlapping set of self-proteins, despite the existence of pathways allowing protein/peptide transfer between cells and despite the fact that a lot of basic cellular components like metabolic enzymes, and structural proteins should be expressed at similar levels in most cells. One reason for this might be the differences in the antigen-processing machinery between the different cell types [13] , [14] , [15] , [16] . To address this question, we compared the source proteins of peptides presented on DCs to that of the DC-depleted fraction (enriched for other thymic APCs, for composition see Supplementary Table S1 and Supplementary Fig. S1 ). In total, we identified 302 peptides originating from 187 different proteins on DCs and 265 peptides from 184 different proteins in the DC-depleted fraction, 71 of which were present in both fractions ( Fig. 3a ). These include proteins such as HLA molecules, histones, proliferating cell nuclear antigen, actin, pyruvate kinase, serum albumin and β2 microglobulin. Although, ~1/3 of the protein pool was shared between DCs and non-DC cells, the majority of the identified proteins were unique for each group, supporting the idea that different thymic APCs present different peptides. 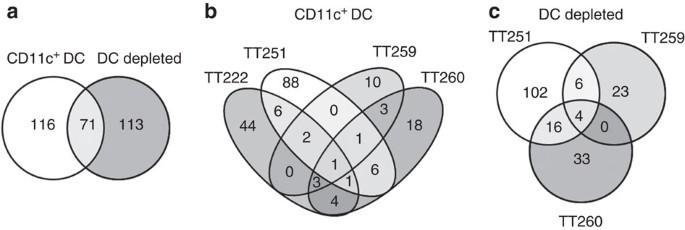Figure 3: Inter-individual variation in presentation of peptides from different source proteins presented by MHC I and II. The diagrams depict the number of different source proteins identified in the different cell preparations as well as overlap between samples. (a) Overlap of identified proteins between mDC and mDC-depleted (enriched for other APC) fractions (individual donors taken together). Inter-individual variations of proteins presented on (b) DC of four different donors and (c) DC-depleted fractions of three individuals, respectively. Figure 3: Inter-individual variation in presentation of peptides from different source proteins presented by MHC I and II. The diagrams depict the number of different source proteins identified in the different cell preparations as well as overlap between samples. ( a ) Overlap of identified proteins between mDC and mDC-depleted (enriched for other APC) fractions (individual donors taken together). Inter-individual variations of proteins presented on ( b ) DC of four different donors and ( c ) DC-depleted fractions of three individuals, respectively. Full size image Data from whole thymus indicated a large degree of variability of the source proteins from which peptides were presented in different donors ( Supplementary Fig. S2 ), probably partially due to differences in HLA-binding preferences and protein expression. Quantitative differences in expression levels of individual MHC–peptide complexes might also play a role as our experimental approach preferentially detects high abundance peptides, especially when source material is limiting. To exclude the possibility that the limited overlap observed was due to issues of technical reproducibility rather than bona fide biological variability, we performed extensive validation experiments which showed that technical reproducibility was in the order of 85%, while the overlap between samples derived from different donors was much lower ( Supplementary Fig. S3 ), demonstrating that the differences observed were indeed due to biological, and not technical, variability. To clarify whether this variability was also observed for the self-proteins directly involved in negative selection of T cells, we compared the source proteins of the peptides eluted from thymic DCs from different donors ( Fig. 3b ). Of the 187 proteins whose peptides were presented by mDCs, only 27 were detected in more than one donor, and only one (HLA-DRB1) was shared by the four individual thymic DC samples. Peptides from seven proteins (HLA-DRA, serum albumin, tubulin β 2 A chain, serine/threonine-protein phosphatase PP1, astrocytic phosphoprotein PEA-15, bax inhibitor 1, signal transducer and activator of transcription 1-α/β) could be detected in three out of four DC samples, but peptides from the vast majority of proteins (160) were only detected in one sample, reflecting a high inter-individual variability in the peptide matrix for negative selection. A similar picture is observed in the DC-depleted-derived peptide pool ( Fig. 3c ). To further explore the differences between the HLA ligandome of DCs and non-DCs, we directly compared the source proteins ( Fig. 4a ) and the protein-derived peptides ( Fig. 4b ) that are present on the respective fractions from the same donors, eliminating the contribution of HLA-binding preference to peptide variability between fractions. Interestingly, only about a fifth of the detected proteins were presented by both DC and non-DC APCs, and for donor TT259 the overlap was even smaller. In summary, we demonstrate a high inter-individual variability of the MHC ligandome and furthermore, our results agree with the notion that different, but overlapping spectra of self-proteins on different thymic APCs results in partially non-redundant contributions of different APCs to negative selection. 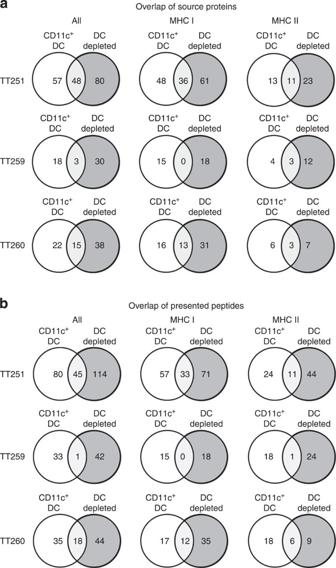Figure 4: Comparison of mDC and non-mDC fractions in each donor. Overlap of (a) source proteins and (b) presented peptides between mDC and mDC-depleted cells in three individual thymi. Figure 4: Comparison of mDC and non-mDC fractions in each donor. Overlap of ( a ) source proteins and ( b ) presented peptides between mDC and mDC-depleted cells in three individual thymi. Full size image T-cell epitopes linked to autoimmunity Incomplete representation of the full spectrum of self-proteins (the ‘immunological self’) on MHC molecules of mTECs and DCs will result in a lack of central tolerance to those epitopes that are not displayed, increasing the propensity for autoreactivity among mature T cells in the periphery [1] , [33] . We were therefore particularly interested whether we could identify peptides corresponding to known T-cell epitopes that have been described as targets in human autoimmune diseases. Literature search yielded a number of T-cell autoantigens that were also detectable in our samples ( Table 2 ). The table only includes T-cell autoantigens for which reactivity has been experimentally verified in humans, such as vimentin (rheumatoid arthritis, sarcoidosis) [34] , [35] , ATP synthase (sarcoidosis) [35] , enolase 2 (multiple sclerosis) [36] and heat shock protein 70 (type 1 diabetes mellitus) [37] . For those autoantigens where reactivity against specific epitopes (rather than whole protein) was reported, the epitopes were identical to, or contained within the peptide sequences that we identified in our samples, mostly on DCs. This clearly demonstrates presentation of these epitopes in normal human thymus, which should lead to deletion of autoreactive T cells. We therefore hypothesize that in patients with autoimmune disease, presentation of these epitopes could be impaired, resulting in failure of central tolerance towards these epitopes. Table 2 T-cell autoantigens/epitopes in humans identified in different thymus samples. Full size table Tumour-associated antigens in the thymus Central tolerance is a double-edged sword. Although it protects us from autoimmune disease, it can also impede anti-tumour immunity. It is likely that presentation of self-proteins which tolerize the T-cell repertoire to self-antigens in order to avoid autoimmunity may also negatively impact the ability of T cells to mediate tumour immunity. This prediction has been confirmed by studies demonstrating the expression of tumour-associated antigens, including differentiation antigens and cancer-germline antigens, in human mTECs [38] , and moreover, expression of the human carcinoembryonic antigen (CEA), in mTECs of transgenic mice induces central tolerance [39] . A thorough literature search on natural MHC ligand repertoires in tumours revealed that a significant number of the MHC-bound peptides detected in our experiments are also found to be (over)presented in renal cell carcinomas [40] , [41] or other disease tissues ( Supplementary Data 2 ), including the SET nuclear oncogene and APOL1. Our findings provide an explanation why only low-avidity T cells against many cancer-associated antigens are present in the periphery [42] , as presentation of tumour-associated antigens by negatively selecting cells of the thymus should result in the deletion of high-avidity T cells. Therefore, even if they are found to be overexpressed on tumour tissues, they might not be the first choice as a target for immunotherapy. An example is p53, a tumour suppressor with a central role in tumour development. Here, we detected a p53-derived peptide presented on MHC I on DCs ( Supplementary Data 1 and 2 ), which should lead to thymic deletion of p53-specific CD8 + T cells. This is in line with a recent ovarian cancer study describing the lack of spontaneous p53-specific CD8 + , but not CD4 + -specific T-cell responses in healthy donors and patients with high antibody titres against p53 (ref. 43 ). In summary, we provide here the first characterization of the peptide repertoire presented by MHC molecules in the healthy human thymus in vivo with a focus on those epitopes presented by mDCs that are important for negative selection. Interestingly, both known autoantigens as well as tumour-associated antigens were detected. We observed a high degree of inter-individual variability between donors that can in part be explained by differences in HLA type but might also be partially due to differences in protein expression. Furthermore, mDCs and non-mDC APCs present different, only partially overlapping sets of peptides, probably due to differences both in self-protein expression as well as differences in their antigen-processing machinery [13] , [15] . Although our data contribute to answer the long-standing question of which peptides are physiologically involved in T-cell selection in the human thymus, many issues still remain to be addressed before we fully understand the process of central tolerance. For example, analysis of ligands derived from isolated mTECs or cTECs as well as low abundance ligands presented by DCs is currently limited by available technology. For this reason, the data presented here are from mDCs only, and do not include ligands from isolated mTECs, which also contribute to central tolerance. Another question that remains to be addressed is whether the thymic ligandome changes considerably during the lifetime of an individual. For obvious reasons it will be difficult to answer this question experimentally in humans, but some previous studies suggest that variation is likely to occur. Thymic DCs and mTECs have a half-life of about 2–3 weeks and at least for mTECs, considerable differences in tissue-restricted antigen expression between different cells have been described [44] . Our and other data support the idea that thymic DCs sample the blood stream for proteins, and peripheral DCs can take up antigens, migrate to the thymus and delete the corresponding T cells [8] , [12] . Changes in the periphery would therefore be expected to impact on the peptides presented in the thymus. Our data should pave the way for a comprehensive understanding of central tolerance and might one day help to improve the design of therapeutic interventions such as cancer vaccines. The expression of ligands derived from tumour-associated antigens on thymic APCs highlights the need for a more systematic analysis of potential cancer vaccine candidates, employing our data to preselect or exclude antigens from the growing list of candidates in future vaccine trials. Thymic samples Normal human thymus samples were obtained from children undergoing corrective cardiac surgery (Department of Cardiac Surgery, University of Tübingen, Germany) after parents’ informed consent and approval by the Institutional Review Board of the Medical Faculty of the University of Tübingen. For details of donors see Table 3 . Table 3 Age, gender and HLA typing of thymus tissue donors included in this study. Full size table Genotyping of thymic tissues DNA for HLA genotyping was extracted from thymus tissue using the QIAamp DNA Blood Mini kit (Qiagen). Low-resolution HLA typing was performed by the Institute for Clinical and Experimental Transfusion Medicine (IKET), University of Tübingen, Germany. Isolation of thymic DCs mDCs were isolated from thymus tissue after mechanical and enzymatic disruption (collagenase (1 mg ml −1 ) and DNase (50 μg ml −1 , both from Roche), at 37 °C, two to three times for 30–45 min) [14] . APCs were enriched from the resulting single-cell suspension by Percoll gradient centrifugation (density: 1.07 g ml −1 , 30 min, 3,500 g, 4 °C) and DCs were isolated by magnetic beads (CD11c-PE and anti-PE beads, Miltenyi Biotec) from the low-density fraction following the manufacturer’s instructions. Both the positive (DC) and negative (DC-depleted) fractions (for composition see Supplementary Table S1 and Supplementary Fig. S1 ) were collected. A summary of the workflow is given in Fig. 1 . FACS Analysis Single-cell suspensions from whole thymus, the APC-enriched fraction after Percoll, DC and DC-depleted fractions were stained with antibodies against HLA–DR (PerCP, 307628, 1:50), CD19 (FITC, 302205, 1:20), CD14 (APC, 301807, 1:50), CD45RA (FITC, 304105, 1:10), CD123 (PE/Cy7, 306009, 1:10), (all from Biolegend), CD45 (PB, PB986, 1:10, DAKO), BDCA-4 (PE, 130-090-533, 1:10), CD11c (PE, 130-092-411, 1:10), EpCAM (APC, 130-091-254, 1:10, from Miltenyi Biotec), CDR2 (1:50, Bruno Kyewski, DKFZ, Heidelberg; labelled with Alexa488 using the Alexa Fluor 488 Protein Labelling kit from Molecular Probes according to manufacturer’s instructions). mDCs were gated as CD11c + , B cells were gated as CD19 + , pDCs as CD45RA + BDCA-4 + , monocytes as CD14 + , mTEC and cTEC as CD45 lo-neg EpCAM hi or CD45 lo-neg EpCAM lo CDR2 + , respectively. Elution of MHC ligands MHC-bound peptides were isolated using antibodies L234 (HLA–DR) and W6/32 (pan-HLA class I) [45] , [46] . We have also published a detailed step-by-step protocol of this procedure [45] . Frozen-cell pellets or tissue pieces were lysed with 0.6% CHAPS with protease inhibitors in PBS, stirring for 2 h at 4 °C. The resulting lysate was ultrasonicated, and debris pelleted by centrifugation (4,000 g for 20 min, followed by ultracentrifugation at 40,000 r.p.m. for 1 h). The supernatant was clarified by ultrafiltration (0.2 μm pore size, Sartolab P plus, Sartorius) and peptide–MHC complexes were isolated from the supernatant by affinity chromatography (antibodies L234 (MHC II) or W6/32 (MHC I) coupled to CNBr-Sepharose, overnight, 4 °C). Bound MHC–peptide complexes were eluted with 0.1% TFA. Eluted peptides were separated from MHC proteins by centrifugation though a filter with a MW cutoff of 10 kDa and analysed by LC-MS/MS. Identification of MHC ligands Nanoscale liquid chromatography of MHC ligands was performed with a Waters NanoAcquity UPLC system equipped with a 75 μm × 150 mm BEH C18 reversed phase column and a 2.6-μl PEEKSIL-sample loop (SGE, Darmstadt, Germany). The aqueous mobile phase (mobile phase A) was H 2 O with 0.1% formic acid. The organic mobile phase (mobile phase B) was 0.1% formic acid in acetonitrile. Samples (2.6 μl injection) were loaded onto the column in direct injection mode with 3% mobile phase B for 15 min at 400 nl min −1 , followed by an additional 10 min wash (3% B) for 10 min at 300 nl min −1 . Peptides were eluted from the column with a gradient from 3–35% mobile phase B over 120 min at 300 nl min −1 followed by a 20-min rinse of 80% mobile phase B. The column was immediately re-equilibrated at initial conditions (3% mobile phase B) for 20 min. [Glu 1 ] fibrinopeptide was used as lockmass at 500 fmol μl −1 . Lockmass solution was delivered from the auxiliary pump of the NanoAcquity system at 400 nl min −1 to the reference sprayer of the NanoLockSpray source. MS/MS analysis of peptides was performed by using a Waters Q-Tof Premier mass spectrometer operated in V-mode with typical resolving power of R =10.000 in data-dependent acquisition mode, selecting the three most intense precursor ions for fractionation in the collision cell. Fragmentation of the parent ions was achieved by collision with argon atoms. Collision energy was varied from 15–35 eV dependent on precursor ion mass and charge. The integration time for the TOF analyser was 1 s with an interscan delay of 0.1 s. Interpretation of MS/MS fragmentation spectra was carried out manually using MassLynx 4.0 software [47] . For manual peptide identification, sequence tag searches were done using Mascot 2.0 software (peptide and MS/MS tolerance, 0.2 Da; National Center for Biotechnology Information non-redundant (NCBInr) database updated monthly and restricted for search to human entries), and relevant hits were assessed manually and not by evaluation of the Mascot score. Criteria for manual identification were: a reasonable interpretation of at least 95% of all fragment peaks, complete sequence coverage with MS/MS fragments, and signal intensities of fragment ion peaks that match breakage probabilities of the respective sequence. The obtained peptide sequences were assigned to source proteins using the BLAST algorithm and further bioinformatics analysis [48] , [49] was performed. The MHC class I and MHC class II ligands in different thymic cell preparations were assigned to subcellular compartments or functional categories according to Gene Ontology annotations ( www.geneontology.org ). In cases where this search yielded no or incomplete information, annotation was performed manually based on information from WoLF PSORT [48] (wolfpsort.org), SubLoc [49] ( www.bioinfo.tsinghua.edu.cn/SubLoc/ ), SwissProt and published literature. Source proteins were then grouped to the classical MHC I (cytosolic, nuclear) or MHC II pathway (extracellular, vesicular and cell membrane), the mitochondrial or ER compartment. To facilitate interpretation of data for biological function, related subcategories were grouped together, for example, ‘signalling’, ‘cell–cell signalling’ and ‘signal transduction’ were grouped together as ‘signalling’. All peptides were assigned to a specific HLA allotype by taking the HLA type of the patient into consideration as well as known binding motifs of different allotypes [50] . Peptides were assigned to the presenting HLA molecule by comparison of their anchor amino acids with known HLA allele-specific peptide motifs. In order to carry out an automated, reproducible assignment to the correct HLA allotype, all peptide sequences were subjected to epitope prediction using the database SYFPEITHI (ref. 50 ) ( www.syfpeithi.de ), evaluating the preferential binding to one of the HLA allotypes defined by HLA typing. SYFPEITHI calculates scores according to the preferred amino acids in each sequence position. Peptides receiving more than the half-maximal score for a given HLA molecule were assigned to the respective molecule. It has to be noted that ligands of different HLA molecules may achieve different maximal scores. The maximal scores are 44 for HLA-A*03, 44 for HLA-A*26, 29 for HLA-A*31, 37 for HLA-A*32, 33 for HLA-B*07, 30 for HLA-B*38 and 38 for HLA-B*51. If epitope prediction was not possible by the web version of SYFPEITHI, an in-house version with extended options was used. This was the case for predictions of HLA-A*31 and HLA-A*32 ligands and for rarely occurring peptide lengths (8 mer, 11 mer) of other HLA allotypes. Reproducibility analysis For method validation and reproducibility analysis, MHC I peptides from PBMC of healthy volunteers were isolated and technical replicates performed. For statistical analysis of the intra-sample (that is, technical) reproducibility, the overlaps of every conceivable pair of technical replicates were calculated for one randomly selected sample. For the assessment of inter-individual variability we analysed the overlaps of HLA ligand source proteomes of five healthy volunteer PBMC samples. We performed comprehensive overlap analysis of all five samples. For the statistical analysis of inter-individual variability, paired overlap analyses of all 10 possible combinations of source proteomes were performed. The two populations (technical replicate overlaps versus inter-individual overlaps) were compared using a two-sided, unpaired Student’s t -test not assuming equal standard deviations ( Supplementary Fig. S3 ). How to cite this article: Adamopoulou, E. et al . Exploring the MHC-peptide matrix of central tolerance in the human thymus. Nat. Commun. 4:2039 doi: 10.1038/ncomms3039 (2013).